The miR-363-GATA6-Lgr5 pathway is critical for colorectal tumourigenesis Aberrant activation of Wnt signalling results in colorectal tumours. Lgr5 is specifically expressed in stem cells of the intestine and has an essential role in maintaining tissue homeostasis. Lgr5-positive stem cells are responsible for the intestinal adenoma initiated by mutations in adenomatous polyposis coli. Furthermore, Lgr5 interacts with R-spondins and thereby activates Wnt signalling. However, the function of Lgr5 in colorectal tumourigenesis is unclear. Here we show that LGR5 is required for the tumourigenicity of colorectal cancer cells. We show that the transcription factor GATA6 directly enhances the expression of LGR5. We further demonstrate that GATA6 is upregulated in colorectal cancer cells due to the downregulation of miR-363, which directly targets GATA6. Moreover, we show that overexpression of miR-363 suppresses the tumourigenicity of colorectal cancer cells. These results suggest that the miR-363-GATA6-LGR5 pathway is critical for colorectal tumourigenesis and would be a promising target for the treatment of colorectal cancer. LGR5, also known as GPR49, is a member of the leucine-rich repeat containing G-protein-coupled receptors (LGRs) and is known as a target of Wnt signalling [1] . Phylogenetic analysis indicates that there are three LGR subgroups: LGR1~3, LGR4~6 and LGR7 and LGR8. The ligands for LGR1~3 are follicle-stimulating hormone, thyroid-stimulating hormone and luteinizing hormone, respectively [2] . The ligands for LGR7 and LGR8 are small heterodimeric peptides with homology to insulin, including the pregnancy hormone relaxin and insulin-like 3 (refs 3 , 4 ). Furthermore, recent studies have shown that Lgr4 and Lgr5 are associated with the Frizzled/Lrp Wnt receptor complex and R-spondins function as their ligands to regulate Wnt signalling [5] , [6] , [7] . LGR5 null mice exhibit neonatal lethality because of ankyloglossia [8] . It has been reported that two types of intestinal stem cells are located at the crypt bottoms: the highly proliferating LGR5 + crypt base columnar cells [9] and the quiescent Bmi-1 + and Hopx + DNA-label retaining cells (LRCs) at position +4 (refs 10 , 11 , 12 ). LGR5-positive stem cells can differentiate into all types of intestinal epithelial cell lineages [9] . When Lgr5 + stem cells are experimentally ablated, LRCs can serve as an alternative stem cell pool [11] . It has also been shown that these two types of cells can be interconverted [12] . More recently, it has been reported that the cycling Lgr5 + stem cells generate LRCs and that the quiescent LRCs are destined to differentiate into Paneth and enteroendocrine cells but can reaquire stem cell properties when the tissue is injured [13] . Furthermore, it has been reported that LGR5 also marks the cycling and long-lived hair follicle stem cells and stomach stem cells as well as the intestinal stem cells [14] , [15] . In all of these tissues, Wnt signalling plays an important role in cell proliferation and tissue homeostasis. LGR5 has been used as a stem cell marker of tissues where the regulation by Wnt signalling has a critical role. In addition, LGR5 has been reported to be upregulated in some cancer tissues, such as basal cell carcinomas, hepatocelluar carcinomas, ovarian tumours and colorectal tumours [16] , [17] . It has also been reported that Lgr5-positive intestinal stem cells are the cells of origin of adenoma initiated by mutations in adenomatous polyposis coli (APC). The members of the GATA family of zinc finger transcription factors play important roles in the development, regulation of differentiation and control of cell proliferation and movement. In mammals, the GATA family is composed of six members, typically divided into two subfamilies based on location, structure and function (GATA-1/2/3 and GATA-4/5/6). GATA-4, -5 and -6 are found mainly in the heart and endoderm-derived tissues, including the liver, lungs, pancreas, stomach and intestines [18] . Furthermore, it has been reported that GATA6 is expressed in proliferating cells in the intestinal crypts and is required for crypt cell proliferation and migration [19] , [20] . Targeted inactivation of the GATA6 gene in mice causes early embryonic lethality due to the lack of endoderm differentiation [21] , [22] , [23] . In the present study, we show that LGR5 is required for the tumourigenicity of colorectal cancer cells. Furthermore, we demonstrate that downregulation of miR-363 results in upregulation of GATA6, which in turn induces LGR5 to promote colorectal cancer. Taken together, these results suggest that the miR-363-GATA6-LGR5 pathway is critical for colorectal tumourigenesis. Lgr5 is required for tumorigenicity of colon cancer cells To clarify the importance of Lgr5 in colorectal tumourigenesis, we infected colon cancer DLD-1 or HT29 cells with a lentivirus expressing an small hairpin RNA (shRNA) against Lgr5. When the stably expressing cells were transplanted into nude mice, cell growth was significantly retarded compared with cells infected with a control lentivirus ( Fig. 1a–d ). Thus, Lgr5 may be required for the tumourigenicity of these colorectal cancer cells. In addition, we observed no histological differences between DLD-1 tumours developed from control or Lgr5-knockdown cells ( Supplementary Fig. 1a ). We also found no differences in the expression of cell lineage markers, including lysozyme staining of Paneth cell granules, periodic acid Schiff staining of mucin production in goblet cells and alkaline phosphatase staining of enterocytes ( Supplementary Fig. 1b ). Colony formation assays with DLD-1 cells in soft agar showed that knockdown of Lgr5 caused a significant reduction in clonogenicity ( Fig. 1e ). However, knockdown of Lgr5 did not affect the growth of DLD-1 cells ( Fig. 1f ). Thus, the effect of Lgr5 knockdown on tumourigenicity may not be simply ascribed to cell cycle arrest or apoptosis. 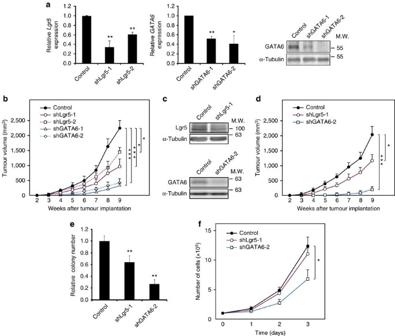Figure 1: Lgr5 and GATA6 are required for the tumourigenicity of colorectal tumor cells. (a) qRT–PCR (left and middle) and immunoblotting (right) analyses of Lgr5 and GATA6 in DLD-1 cells that were infected with a lentivirus expressing an shRNA targeting Lgr5 or GATA6. Two distinct shRNAs targeting Lgr5 or GATA6 were used. Results are expressed as the means±s.d. of three independent experiments.GAPDHwas used as an internal control. α-Tubulin was used as a loading control. *P<0.05 and **P<0.01, Student’st-test. (b) DLD-1 cells infected with a lentivirus expressing an shRNA against Lgr5 or GATA6 or control shRNA were subcutaneously injected into nude mice (n=8 per group). Results are expressed as the mean±s.e.m. *P<0.05 and ***P<0.001, Student’st-test. (c) Suppression of Lgr5 or GATA6 expression in HT29 cells by shRNAs. Cells were infected with a lentivirus expressing an shRNA targeting Lgr5 or GATA6. Lysates prepared from infected cells were analysed by immunoblotting with anti-Lgr5 and anti-GATA6 antibodies. Anti-α-tubulin antibody was used as a control. (d) HT29 cells infected with a lentivirus expressing an shRNA against Lgr5 or GATA6, or control shRNA, were subcutaneously injected into nude mice (n=8 per group). Results are expressed as the mean±s.e.m. *P<0.05 and ***P<0.001, Student’st-test. (e) Knockdown of Lgr5 or GATA6 inhibit colony formation in soft agar. DLD-1 cells were infected with a lentivirus expressing a control or shRNA targeting Lgr5 or GATA6 and subjected to colony formation assays in soft agar. The number of colonies is shown as the relative number. Results are expressed as the mean±s.e.m. of three independent experiments. **P<0.01, Student’st-test. (f) Knockdown of Lgr5, unlike GATA6, does not affect the proliferation of DLD-1 cells under adherent conditions. DLD-1 cells infected with a lentivirus expressing an shRNA targeting Lgr5 or GATA6, or control shRNA, were plated (day 0) and cell numbers were counted every 24 h. The means±s.d. of three independent experiments are shown. *P<0.05, Student’st-test. Figure 1: Lgr5 and GATA6 are required for the tumourigenicity of colorectal tumor cells. ( a ) qRT–PCR (left and middle) and immunoblotting (right) analyses of Lgr5 and GATA6 in DLD-1 cells that were infected with a lentivirus expressing an shRNA targeting Lgr5 or GATA6. Two distinct shRNAs targeting Lgr5 or GATA6 were used. Results are expressed as the means±s.d. of three independent experiments. GAPDH was used as an internal control. α-Tubulin was used as a loading control. * P <0.05 and ** P <0.01, Student’s t -test. ( b ) DLD-1 cells infected with a lentivirus expressing an shRNA against Lgr5 or GATA6 or control shRNA were subcutaneously injected into nude mice ( n =8 per group). Results are expressed as the mean±s.e.m. * P <0.05 and *** P <0.001, Student’s t -test. ( c ) Suppression of Lgr5 or GATA6 expression in HT29 cells by shRNAs. Cells were infected with a lentivirus expressing an shRNA targeting Lgr5 or GATA6. Lysates prepared from infected cells were analysed by immunoblotting with anti-Lgr5 and anti-GATA6 antibodies. Anti-α-tubulin antibody was used as a control. ( d ) HT29 cells infected with a lentivirus expressing an shRNA against Lgr5 or GATA6, or control shRNA, were subcutaneously injected into nude mice ( n =8 per group). Results are expressed as the mean±s.e.m. * P <0.05 and *** P <0.001, Student’s t -test. ( e ) Knockdown of Lgr5 or GATA6 inhibit colony formation in soft agar. DLD-1 cells were infected with a lentivirus expressing a control or shRNA targeting Lgr5 or GATA6 and subjected to colony formation assays in soft agar. The number of colonies is shown as the relative number. Results are expressed as the mean±s.e.m. of three independent experiments. ** P <0.01, Student’s t -test. ( f ) Knockdown of Lgr5, unlike GATA6, does not affect the proliferation of DLD-1 cells under adherent conditions. DLD-1 cells infected with a lentivirus expressing an shRNA targeting Lgr5 or GATA6, or control shRNA, were plated (day 0) and cell numbers were counted every 24 h. The means±s.d. of three independent experiments are shown. * P <0.05, Student’s t -test. Full size image GATA6 upregulates Lgr5 expression in colorectal cancer cells To identify transcription factors that are involved in the regulation of Lgr5 expression in colon tumours, we searched for transcription factor-binding motifs present in the promoter region of Lgr5 . We selected 104 candidate transcription factors and examined whether small interfering RNA (siRNA)-mediated knockdown of any of these affected Lgr5 expression in DLD-1 cells. Among these genes, knockdown of GATA6 caused the most significant decrease in Lgr5 expression ( Fig. 2 ). 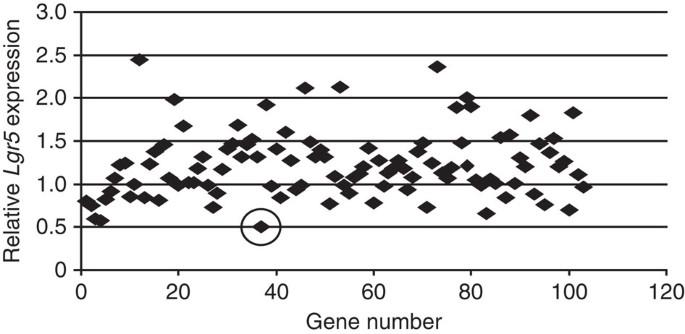Figure 2: siRNA screen for transcription factors involved in the regulation of Lgr5 expression. DLD-1 cells were transfected with siRNA and the expression levels ofLgr5mRNA were assessed by qRT–PCR. GAPDH was used as an internal control. The black circle indicates the data obtained from cells transfected with siRNA targeting GATA6. Figure 2: siRNA screen for transcription factors involved in the regulation of Lgr5 expression. DLD-1 cells were transfected with siRNA and the expression levels of Lgr5 mRNA were assessed by qRT–PCR. GAPDH was used as an internal control. The black circle indicates the data obtained from cells transfected with siRNA targeting GATA6. Full size image GATA6 is a zinc finger transcription factor that is required for the proliferation, development and specific gene regulation of the gastrointestinal tract and other tissues [24] , [25] , [26] . GATA6 has also been reported to be involved in colorectal tumour invasion and in the conversion of Barrett metaplasia to adenocarcinoma [27] , [28] . Furthermore, GATA6 is known to be expressed in the proliferative crypt compartment of the small intestine, similar to Lgr5, although expression is found elsewhere as well [19] , [25] . We therefore focused our analyses on GATA6. We confirmed that knockdown of GATA6 reduced the amount of Lgr5 mRNA in DLD-1 cells ( Fig. 3a ). Consistent with this result, overexpression of GATA6 resulted in the upregulation of Lgr5 expression ( Fig. 3b ). These results suggest that GATA6 regulates Lgr5 expression in colorectal cancer cells. 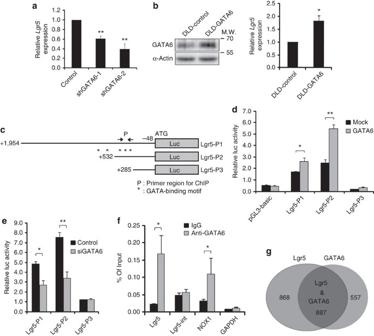Figure 3: GATA6 upregulates Lgr5 expression in colorectal cancer cells. (a) qRT–PCR analysis of Lgr5 expression in DLD-1 cells infected with a lentivirus expressing shRNA targeting GATA6. Results are expressed as the means±s.d. of three independent experiments. **P<0.01, Student’st-test. (b) Overexpression of GATA6 upregulatesLgr5expression. Cell lysates from DLD-1 cells infected with a control or GATA6 expressing lentivirus were subjected to qRT–PCR analysis. Results are expressed as the means±s.d. of two independent experiments. *P<0.05, Student’st-test. (c) Schematic diagrams of reporter constructs used for luciferase assays. Fragments of theLgr5promoter were cloned upstream of the luciferase (luc) gene: Lgr5-P1 (from +1,954 to −48), Lgr5-P2 (from +532 to −48) and Lgr5-P3 (from +285 to −48). The potential GATA sites are indicated by asterisks and the primer region for ChIP assays are represented as P. (d) RKO cells were co-transfected with mock or HA-tagged GATA6 vector and reporter constructs containingLgr5promoter sequences and were subjected to luciferase assays. pRL-TK vector was used as an internal control. Results are expressed as the means±s.d. of three independent experiments. *P<0.05 and **P<0.01, Student’st-test. (e) DLD-1 cells that had been transfected with siRNA targeting GATA6 or with control siRNA were transfected with Lgr5 reporter constructs and subjected to luciferase assays. Results are shown as the means±s.d. of three independent experiments. *P<0.05 and **P<0.01, Student’st-test. (f) ChIP assays were performed on DLD-1 cells using an anti-GATA6 or anti-rabbit IgG antibody. The promoter region ofLgr5was amplified. The promoter regions ofNOX1andGAPDHwere used as positive and negative controls, respectively. Results are expressed as the means of percentage of input ±s.d. of three independent experiments. *P<0.05, Student’st-test. (g) Venn diagram showing the overlap between genes downregulated by knockdown of Lgr5 and those downregulated by knockdown of GATA6. TheP-value for the significance of the overlap is 0 as determined by hypergeometric distribution. Figure 3: GATA6 upregulates Lgr5 expression in colorectal cancer cells. ( a ) qRT–PCR analysis of Lgr5 expression in DLD-1 cells infected with a lentivirus expressing shRNA targeting GATA6. Results are expressed as the means±s.d. of three independent experiments. ** P <0.01, Student’s t -test. ( b ) Overexpression of GATA6 upregulates Lgr5 expression. Cell lysates from DLD-1 cells infected with a control or GATA6 expressing lentivirus were subjected to qRT–PCR analysis. Results are expressed as the means±s.d. of two independent experiments. * P <0.05, Student’s t -test. ( c ) Schematic diagrams of reporter constructs used for luciferase assays. Fragments of the Lgr5 promoter were cloned upstream of the luciferase (luc) gene: Lgr5-P1 (from +1,954 to −48), Lgr5-P2 (from +532 to −48) and Lgr5-P3 (from +285 to −48). The potential GATA sites are indicated by asterisks and the primer region for ChIP assays are represented as P. ( d ) RKO cells were co-transfected with mock or HA-tagged GATA6 vector and reporter constructs containing Lgr5 promoter sequences and were subjected to luciferase assays. pRL-TK vector was used as an internal control. Results are expressed as the means±s.d. of three independent experiments. * P <0.05 and ** P <0.01, Student’s t -test. ( e ) DLD-1 cells that had been transfected with siRNA targeting GATA6 or with control siRNA were transfected with Lgr5 reporter constructs and subjected to luciferase assays. Results are shown as the means±s.d. of three independent experiments. * P <0.05 and ** P <0.01, Student’s t -test. ( f ) ChIP assays were performed on DLD-1 cells using an anti-GATA6 or anti-rabbit IgG antibody. The promoter region of Lgr5 was amplified. The promoter regions of NOX1 and GAPDH were used as positive and negative controls, respectively. Results are expressed as the means of percentage of input ±s.d. of three independent experiments. * P <0.05, Student’s t -test. ( g ) Venn diagram showing the overlap between genes downregulated by knockdown of Lgr5 and those downregulated by knockdown of GATA6. The P- value for the significance of the overlap is 0 as determined by hypergeometric distribution. Full size image To clarify the mechanisms underlying GATA6-mediated upregulation of Lgr5, we monitored expression of reporter constructs in which various fragments of the Lgr5 promoter region (Lgr5-P1, -P2 and -P3 in Fig. 3c ) were inserted upstream of the luciferase gene. These promoter regions contain 5, 3 or no GATA-binding sites, respectively. When transfected into RKO cells, the activities of the Lgr5-P1 and -P2 reporters, but not the Lgr5-P3 reporter, were significantly enhanced by coexpression of GATA6 ( Fig. 3d ). Consistent with these results, knockdown of GATA6 using siRNA reduced the activities of LGR5-P1 and -P2 ( Fig. 3e ). To confirm that GATA6 transactivates Lgr5 directly, we performed chromatin immunoprecipitation (ChIP) assays on DLD-1 cells using anti-GATA6 antibody. We detected GATA6 binding to the DNA fragment shown in Fig. 3c , which contains three GATA motifs ( Fig. 3f ). The promoter regions of NOX1 and GAPDH were used as positive and negative controls, respectively. Although a previous in vitro analysis by electrophoresis mobility shift assay indicated that GATA6 binds to GATA sites in the first intron of the Lgr5 gene [29] , our ChIP assays with DLD-1 cells did not detect GATA6 binding to this region (Lgr5-int). Taken together, these results suggest that GATA6 directly upregulates the transcription of Lgr5 by binding to GATA motifs located in its promoter region. We next investigated the gene expression profiles of DLD-1 cells in which Lgr5 or GATA6 expression was suppressed. DNA microarray analyses revealed that the expression profile of GATA6-knockdown cells closely resembled that of LGR5-knockdown cells ( Fig. 3g ), consistent with the idea that Lgr5 is a direct target gene of GATA6. GATA6 is required for tumorigenicity of colon cancer cells To determine the roles of GATA6 in colorectal tumorigenesis, we infected DLD-1 or HT29 cells with a lentivirus expressing an shRNA targeting GATA6 and examined their tumourigenic activities. When implanted into nude mice, the growth of these cells was markedly impaired compared with the parental cells ( Figs 1a–d and 4a ). Colony formation assays with DLD-1 cells in soft agar showed that knockdown of GATA6 caused a significant reduction in clonogenicity ( Fig. 1e ). We also found that knockdown of GATA6 in DLD-1 cells led to a significant decrease in cell proliferation under adherent cell culture conditions ( Fig. 1f ). Furthermore, we found that overexpression of Lgr5 partially restored the colony formation activity and tumourigenicity of DLD-1 cells in which GATA6 had been knocked down ( Fig. 4b–e ). These results indicate that the GATA6-Lgr5 pathway plays an important role in colorectal tumorigenesis. 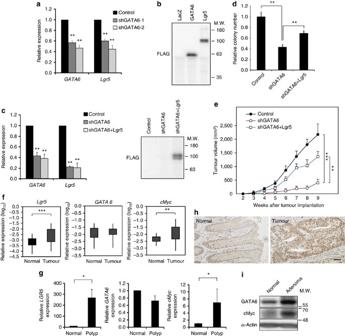Figure 4: GATA6 is required for the tumourigenicity of colorectal tumour cells. (a) qRT–PCR analysis ofGATA6andLgr5expression in DLD-1 tumours from nude mice. DLD-1 cells infected with a lentivirus expressing an shRNA targeting GATA6 were injected into nude mice. Results are expressed as the means±s.d. of three independent experiments. **P<0.01, Student’st-test. (b) Expression of lentiviral GATA6 and Lgr5 in DLD-1 cells. Lysates from cells infected with a lentivirus encoding FLAG-tagged GATA6 or Lgr5 were immunoprecipitated with antibodies against FLAG, and then analysed by immunoblotting with anti-FLAG antibody. A lentivirus encoding LacZ was used as a control. (c) Expression of Lgr5 in DLD-1 cells in which GATA6 had been knocked down. (Left) qRT–PCR analysis of GATA6 and Lgr5 expression in DLD-1 cells infected with a lentivirus expressing an shRNA targeting GATA6 and/or a lentivirus expressing FLAG-tagged Lgr5. Primers for endogeneous Lgr5 were designed to target its 3′-UTR. Results are expressed as the means±s.d. of three independent experiments. (right) Lysates from these cells were subjected to immunoprecipitation with anti-FLAG antibody followed by immunoblotting with anti-FLAG antibody. **P<0.01, Student’st-test. (d,e) Lentiviral expression of Lgr5 restores the colony-forming ability (d) and tumourigenecity (e) of DLD-1 cells in which GATA6 had been knocked down. Transduced cells were subjected to colony formation assays (n=3) in soft agar or injected subcutaneously into nude mice (n=7 per group) and assessed for tumour growth. Results are expressed as the mean±s.e.m. **P<0.01 and ***P<0.001, Student’st-test. (f) The expression of Lgr5, GATA6 and cMyc in human colorectal cancer tissues. Quantitative analysis ofLgr5(left),GATA6(middle) andcMyc(right) mRNA expression in human colon cancerous and corresponding noncancerous tissues by real-time RT–PCR.Lgr5,GATA6andcMycmRNA expression was quantitated as the percentage relative toGAPDHmRNA (n=20–29 pairs). **P<0.01 and ***P<0.001, the Mann–WhitneyU-test. (g) qRT–PCR analysis ofLGR5,GATA6andcMyc.Tissue lysates from adenomas and adjacent normal intestine ofApcMin/+mice were subjected to qRT–PCR with specific primers.GAPDHwas used as an internal control and cMyc was used as a marker of the Wnt pathway activation. Data are expressed as the means±s.d. (n=4–5) *P<0.05, Student’st-test. (h) Immunohistochemical analysis of GATA6 in human colorectal cancer. Paraffin sections of human colorectal cancer tissues and adjacent morphologically normal tissues were immunostained with anti-GATA6 antibody. Scale bar, 50 μm. (i) Immunoblotting analysis of normal and adenoma tissues fromApcMin/+mice with the indicated antibodies. α-Actin and cMyc were used as a loading control and a marker of Wnt pathway activation, respectively. Figure 4: GATA6 is required for the tumourigenicity of colorectal tumour cells. ( a ) qRT–PCR analysis of GATA6 and Lgr5 expression in DLD-1 tumours from nude mice. DLD-1 cells infected with a lentivirus expressing an shRNA targeting GATA6 were injected into nude mice. Results are expressed as the means±s.d. of three independent experiments. ** P <0.01, Student’s t -test. ( b ) Expression of lentiviral GATA6 and Lgr5 in DLD-1 cells. Lysates from cells infected with a lentivirus encoding FLAG-tagged GATA6 or Lgr5 were immunoprecipitated with antibodies against FLAG, and then analysed by immunoblotting with anti-FLAG antibody. A lentivirus encoding LacZ was used as a control. ( c ) Expression of Lgr5 in DLD-1 cells in which GATA6 had been knocked down. (Left) qRT–PCR analysis of GATA6 and Lgr5 expression in DLD-1 cells infected with a lentivirus expressing an shRNA targeting GATA6 and/or a lentivirus expressing FLAG-tagged Lgr5. Primers for endogeneous Lgr5 were designed to target its 3′-UTR. Results are expressed as the means±s.d. of three independent experiments. (right) Lysates from these cells were subjected to immunoprecipitation with anti-FLAG antibody followed by immunoblotting with anti-FLAG antibody. ** P <0.01, Student’s t -test. ( d , e ) Lentiviral expression of Lgr5 restores the colony-forming ability ( d ) and tumourigenecity ( e ) of DLD-1 cells in which GATA6 had been knocked down. Transduced cells were subjected to colony formation assays ( n =3) in soft agar or injected subcutaneously into nude mice ( n =7 per group) and assessed for tumour growth. Results are expressed as the mean±s.e.m. ** P <0.01 and *** P <0.001, Student’s t -test. ( f ) The expression of Lgr5, GATA6 and cMyc in human colorectal cancer tissues. Quantitative analysis of Lgr5 (left), GATA6 (middle) and cMyc (right) mRNA expression in human colon cancerous and corresponding noncancerous tissues by real-time RT–PCR. Lgr5 , GATA6 and cMyc mRNA expression was quantitated as the percentage relative to GAPDH mRNA ( n =20–29 pairs). ** P <0.01 and *** P <0.001, the Mann–Whitney U -test. ( g ) qRT–PCR analysis of LGR5 , GATA6 and cMyc. Tissue lysates from adenomas and adjacent normal intestine of Apc Min/+ mice were subjected to qRT–PCR with specific primers. GAPDH was used as an internal control and cMyc was used as a marker of the Wnt pathway activation. Data are expressed as the means±s.d. ( n =4–5) * P <0.05, Student’s t -test. ( h ) Immunohistochemical analysis of GATA6 in human colorectal cancer. Paraffin sections of human colorectal cancer tissues and adjacent morphologically normal tissues were immunostained with anti-GATA6 antibody. Scale bar, 50 μm. ( i ) Immunoblotting analysis of normal and adenoma tissues from Apc Min/+ mice with the indicated antibodies. α-Actin and cMyc were used as a loading control and a marker of Wnt pathway activation, respectively. Full size image Consistent with previous studies [17] , [27] , we found that Lgr5 mRNA expression was higher in colorectal tumours than in adjacent normal tissues ( Fig. 4f ). We also found that Lgr5 expression was upregulated in intestinal adenomas in Apc Min/+ mice, which are heterozygous for an Apc mutation and spontaneously develop adenomas in the intestine [30] ( Fig. 4g ). By contrast, GATA6 protein, but not its mRNA, was abundantly expressed in human colorectal cancer tissues and intestinal adenomas in Apc Min/+ mice compared with normal tissues ( Fig. 4f–i ). miR-363 regulates GATA6 expression in colon cancer cells It has been shown that microRNAs (miRNAs) function as important post-transcriptional regulators of mRNA expression and/or translation by binding to the 3′untranslated region (UTR) of the cognate mRNA [31] , [32] . The fact that only GATA6 protein, but not its mRNA levels are high in colorectal cancer cells suggests that GATA6 expression is regulated post-transcriptionally. Indeed, we found that knockdown of either Drosha or Dicer, key components of miRNA processing, led to increases in GATA6 protein, but not GATA6 mRNA, and Lgr5 mRNA expression in DLD-1 cells ( Fig. 5a,b ). To identify miRNAs that directly target GATA6 , we performed an in silico search for putative miRNA-binding sites in the 3′-UTR of the human GATA6 mRNA using TargetScan. Among 13 candidates conserved between human and mouse, we focused on miR-363 because its expression was frequently downregulated in human colorectal cancer tissues and intestinal adenomas in Apc Min/+ mice compared with normal tissues ( Fig. 5c,d ). Overexpression of the pre-miR-363, but not the pre-miR-control in DLD-1 cells, led to reductions in GATA6 protein and Lgr5 protein and mRNA levels ( Fig. 5e,f ). We also found that exogenous miR-363 suppresses both GATA6 and Lgr5 expressions in HT29, SW403 and SW948 colon cancer cells. ( Fig. 5g,h ). To confirm that miR-363 regulates GATA6 expression through binding to the seed sequence in GATA6 3′-UTR, we constructed a reporter vector containing the GATA6 3′-UTR region fused to downstream of the luciferase gene driven by the TK promoter (WT 3′-UTR). We also generated a luciferase reporter that contains a mutated miR-363 seed sequence in the GATA6 3′-UTR region (Mut 3′-UTR; Fig. 5i ). Transfection of the pre-miR-363 into DLD-1 cells resulted in decreased luciferase activity from the WT 3′-UTR but not the Mut 3′-UTR construct ( Fig. 5j ). These results suggest that miR-363 has the potential to suppress GATA6 expression through direct binding to the putative miR-363-binding site in the GATA6 3′-UTR region. 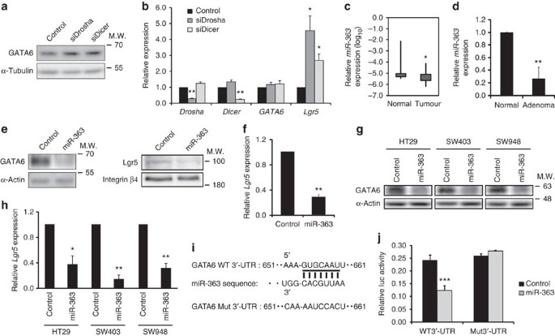Figure 5: miR-363 regulates the expression of GATA6 in colorectal cancer cells. (a,b) Knockdown of Drosha or Dicer increased GATA6 protein levels. DLD-1 cells were transfected with control siRNA or siRNA targeting Drosha or Dicer and subjected to immunoblotting (a) or qRT–PCR (b) analyses using the indicated antibodies and primers, respectively. Results are shown as the means±s.d. of two independent experiments. *P<0.05 and **P<0.01, Student’st-test. (c) The expression of miR-363 is downregulated in human colorectal cancer tissues. Total RNA containing small RNAs from human cancerous tissues and paired normal tissues (n=23) were subjected to qRT–PCR analyses. miR-363 expression was quantitated as the percentage relative toU6mRNA. Box edges and whiskers indicate the 25th/75th and 0th/100th percentiles, respectively. *P<0.05, the Mann–WhitneyU-test. (d) The expression of miR-363 is downregulated in intestinal adenomas inApcMin/+mice. qRT–PCR was performed using total RNA isolated from intestinal adenomas and adjacent normal mucosas inApcMin/+mice (n=4).U6was used as an internal control. Results are expressed as the means±s.d. **P<0.01, Student’st-test. (e,f) Overexpression of miR-363 suppresses both GATA6 and Lgr5 expression. DLD-1 cells were transfected with pre-miR-363 or pre-miR-negative control and subjected to immunoblotting analysis with the indicated antibodies (e) and to qRT–PCR analysis (f). Membrane proteins purified from biotinylated cells with streptavidin-agarose were used for immunoblotting analysis of Lgr5 protein. Integrin β4 was used as a membrane marker. Results are expressed as the means±s.d. of three independent experiments. **P<0.01, Student’st-test. (g,h) Overexpression of miR-363 suppresses both GATA6 and Lgr5 expression in HT29, SW403 and SW948 cells. HT29, SW403 and SW948 cells were transfected with pre-miR-363 or pre-miR-negative control and subjected to immunoblotting analysis with the indicated antibodies (g) and to qRT–PCR analysis (h). Results are expressed as the means±s.d. of three independent experiments. *P<0.05 and **P<0.01, Student’st-test. (i) Predicted duplex sequences between wild-type or mutatedGATA63′-UTR and miR-363. (j) DLD-1 cells were co-transfected with a reporter plasmid and pre-miR-negative control or pre-miR-363 and were subjected to luciferase assays. WT 3′-UTR and Mut 3′-UTR; luciferase reporters containing a wild-type or mutated miR-363 seed sequence in theGATA63′-UTR region, respectively. Each experiment was performed in triplicate, and the results are expressed as the mean±s.d. of three independent experiments. ***P<0.001, Student’st-test. Figure 5: miR-363 regulates the expression of GATA6 in colorectal cancer cells. ( a , b ) Knockdown of Drosha or Dicer increased GATA6 protein levels. DLD-1 cells were transfected with control siRNA or siRNA targeting Drosha or Dicer and subjected to immunoblotting ( a ) or qRT–PCR ( b ) analyses using the indicated antibodies and primers, respectively. Results are shown as the means±s.d. of two independent experiments. * P <0.05 and ** P <0.01, Student’s t -test. ( c ) The expression of miR-363 is downregulated in human colorectal cancer tissues. Total RNA containing small RNAs from human cancerous tissues and paired normal tissues ( n =23) were subjected to qRT–PCR analyses. miR-363 expression was quantitated as the percentage relative to U6 mRNA. Box edges and whiskers indicate the 25th/75th and 0th/100th percentiles, respectively. * P <0.05, the Mann–Whitney U -test. ( d ) The expression of miR-363 is downregulated in intestinal adenomas in Apc Min/+ mice. qRT–PCR was performed using total RNA isolated from intestinal adenomas and adjacent normal mucosas in Apc Min/+ mice ( n =4). U6 was used as an internal control. Results are expressed as the means±s.d. ** P <0.01, Student’s t -test. ( e , f ) Overexpression of miR-363 suppresses both GATA6 and Lgr5 expression. DLD-1 cells were transfected with pre-miR-363 or pre-miR-negative control and subjected to immunoblotting analysis with the indicated antibodies ( e ) and to qRT–PCR analysis ( f ). Membrane proteins purified from biotinylated cells with streptavidin-agarose were used for immunoblotting analysis of Lgr5 protein. Integrin β4 was used as a membrane marker. Results are expressed as the means±s.d. of three independent experiments. ** P <0.01, Student’s t -test. ( g , h ) Overexpression of miR-363 suppresses both GATA6 and Lgr5 expression in HT29, SW403 and SW948 cells. HT29, SW403 and SW948 cells were transfected with pre-miR-363 or pre-miR-negative control and subjected to immunoblotting analysis with the indicated antibodies ( g ) and to qRT–PCR analysis ( h ). Results are expressed as the means±s.d. of three independent experiments. * P <0.05 and ** P <0.01, Student’s t -test. ( i ) Predicted duplex sequences between wild-type or mutated GATA6 3′-UTR and miR-363. ( j ) DLD-1 cells were co-transfected with a reporter plasmid and pre-miR-negative control or pre-miR-363 and were subjected to luciferase assays. WT 3′-UTR and Mut 3′-UTR; luciferase reporters containing a wild-type or mutated miR-363 seed sequence in the GATA6 3′-UTR region, respectively. Each experiment was performed in triplicate, and the results are expressed as the mean±s.d. of three independent experiments. *** P <0.001, Student’s t -test. Full size image The miR-363-GATA6-LGR5 pathway is crucial for tumourigenesis To investigate whether miR-363-mediated suppression of GATA6 expression could decrease the tumourigenicity of colorectal cancer cells, we infected DLD-1 cells with a lentivirus expressing miR-363 to generate DLD-363 cells. Immunoblotting analysis revealed that GATA6 expression was suppressed in DLD-363 cells compared with parental cells infected with control virus ( Fig. 6a ). When subcutaneously inoculated into nude mice, DLD-363 cells showed reduced tumourigenicity compared with control DLD-1 cells ( Fig. 6b ). We also found that DLD-363 cells exhibited decreased colony formation and growth rates compared with DLD-1 cells infected with control virus ( Fig. 6c,d ). Furthermore, we found that overexpression of either GATA6 or Lgr5 could restore the tumourigenicity and colony-forming ability of DLD-363 cells ( Figs 4b and 6b,e,f ). In addition, knockdown of miR-363 resulted in an increase in the levels of GATA6 protein, but not mRNA, and Lgr5 mRNA in human pulmonary arterial endothelial cells (HPAECs), which express significant levels of miR-363 ( Fig. 6g and Supplementary Fig. 2 ). These results suggest that miR-363 inhibits the tumourigenicity of colorectal cancer cells through suppression of GATA6 expression. Thus, the decreased expression of miR-363 in colorectal cancer cells may be responsible for the upregulation of GATA6 and Lgr5, which in turn are required for the tumourigenicity of colorectal cancer cells. 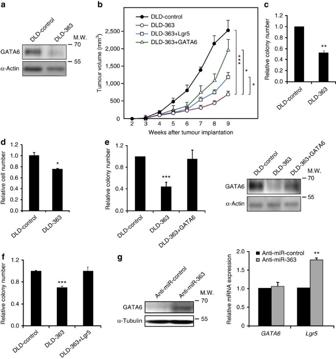Figure 6: miR-363 suppresses the tumourigenicity of colorectal cancer by regulating the expression of GATA6. (a) DLD-1 cells infected with a lentivirus expressing miR-363 (DLD-363) or control virus (DLD-control) were subjected to immunoblotting analysis with the indicated antibodies. Anti-α-actin antibody was used as a control. (b) DLD-control and DLD-363 cells infected with a lentivirus expressing Lgr5 or GATA6 were subcutaneously injected into nude mice (n=8 per group). Results are expressed as the mean±s.e.m. *P<0.05 and ***P<0.001, Student’st-test. (c) DLD-control and DLD-363 cells were subjected to colony formation assays in soft agar. Results are expressed as the mean±s.e.m. of three independent experiments. **P<0.01, Student’st-test. (d) DLD-control and DLD-363 cells were cultured for 3 days and the number of cells was counted. The means±s.d. of three independent experiments are shown. *P<0.05, Student’st-test. (e,f) Overexpression of either GATA6 or Lgr5 restores the colony-forming ability of DLD-363 cells. DLD-363 cells were infected with a lentivirus expressing GATA6 (e, left) or Lgr5 (f). Cell lysates were subjected to immunoblotting analysis with the indicated antibodies (e, right). Anti-α-actin antibody was used as a control. The means±s.d. of triplicate determinations are shown. ***P<0.001, Student’st-test. (g) Inhibition of miR-363 results in an increase in the levels of GATA6 and Lgr5 in HPAECs. Cells were transfected with antisense oligonucleotide against miR-363 and were subjected to immunoblotting analysis with the indicated antibodies (left) or qRT–PCR analysis with the indicated primers (right). The means±s.d. of three independent experiments are shown. **P<0.01, Student’st-test. Figure 6: miR-363 suppresses the tumourigenicity of colorectal cancer by regulating the expression of GATA6. ( a ) DLD-1 cells infected with a lentivirus expressing miR-363 (DLD-363) or control virus (DLD-control) were subjected to immunoblotting analysis with the indicated antibodies. Anti-α-actin antibody was used as a control. ( b ) DLD-control and DLD-363 cells infected with a lentivirus expressing Lgr5 or GATA6 were subcutaneously injected into nude mice ( n =8 per group). Results are expressed as the mean±s.e.m. * P <0.05 and *** P <0.001, Student’s t -test. ( c ) DLD-control and DLD-363 cells were subjected to colony formation assays in soft agar. Results are expressed as the mean±s.e.m. of three independent experiments. ** P <0.01, Student’s t -test. ( d ) DLD-control and DLD-363 cells were cultured for 3 days and the number of cells was counted. The means±s.d. of three independent experiments are shown. * P <0.05, Student’s t -test. ( e , f ) Overexpression of either GATA6 or Lgr5 restores the colony-forming ability of DLD-363 cells. DLD-363 cells were infected with a lentivirus expressing GATA6 ( e , left) or Lgr5 ( f ). Cell lysates were subjected to immunoblotting analysis with the indicated antibodies ( e , right). Anti-α-actin antibody was used as a control. The means±s.d. of triplicate determinations are shown. *** P <0.001, Student’s t -test. ( g ) Inhibition of miR-363 results in an increase in the levels of GATA6 and Lgr5 in HPAECs. Cells were transfected with antisense oligonucleotide against miR-363 and were subjected to immunoblotting analysis with the indicated antibodies (left) or qRT–PCR analysis with the indicated primers (right). The means±s.d. of three independent experiments are shown. ** P <0.01, Student’s t -test. Full size image It has been shown that Lgr5 is a Wnt target gene and is highly expressed in several tumour cell types, including colorectal cancer cells [1] , [16] , [17] , [33] , [34] . We have shown that knockdown of Lgr5 results in a reduction in the tumourigenicity of colorectal cancer cells. This result is consistent with a previous report showing that human immortalized keratinocyte HaCaT cells overexpressing Lgr5 could form tumours when transplanted into immunodeficient mice [16] . Intriguingly, knockdown of Lgr5 caused a significant reduction in clonogenicity of DLD-1 cells, but did not affect their growth under adherent conditions. Thus, the effect of Lgr5 knockdown on tumourigenicity may not simply be ascribed to cell cycle arrest or apoptosis. It is therefore interesting to speculate that these phenotypes might be caused by the loss of stem-like properties. In contrast to our results, it has been reported that Lgr5 suppresses the tumourigenicity of colorectal cancer cell lines carrying a β-catenin mutation [35] . The reason for this difference could be that we used cell lines having APC mutations. However, the precise reasons for this difference remain to be investigated. We found that GATA6 enhances the expression of Lgr5 by directly upregulating its promoter activity in colorectal cancer cells. We also showed that knockdown of GATA6 leads to a significant reduction in the tumourigenicity and colony-forming ability of colorectal cancer cells. Furthermore, we found that overexpression of Lgr5 partially restored the tumourigenicity and colony-forming capacity of colorectal tumour cells in which GATA6 was knocked down. Thus, the GATA6-Lgr5 pathway may be critical for colorectal tumourigenesis. In these experiments, the effects of GATA6 knockdown were more significant than those of Lgr5 knockdown. Furthermore, overexpression of Lgr5 only partially rescued the phenotypes caused by GATA6 knockdown. In addition, we found that knockdown of GATA6, but not of Lgr5 leads to a decrease in the proliferation of DLD-1 cells. These results suggest that GATA6 also has important target genes other than Lgr5. Since GATA6 is highly expressed in the crypt compartment in the intestine [19] , it may also play an essential role in the regulation of Lgr5 expression in intestinal stem cells. Consistent with this notion, it has recently been reported that conditional deletion of GATA6 in intestinal epithelium results in decreased proliferation of crypt progenitor cells and abnormal differentiation of secretary cells [26] . It has been shown that GATA factors interact with transcription factors of various families. For example, the homeodomain protein CDX2, a critical regulator of intestinal homeostasis, plays an important role in intestinal cell proliferation by interacting with GATA6 at active chromatins [25] . Hepatocyte nuclear factor (HNF) family proteins also cooperate with GATA6 to regulate gene expression [36] , [37] . Furthermore, several HNF-binding motifs are present just proximal to the GATA6-binding site in the promoter region of Lgr5 . However, we found that knockdown of CDX2 or HNF family proteins had no significant effect on Lgr5 expression in DLD-1 cells. We found that miR-363 is downregulated in colorectal tumours and that miR-363 has the potential to suppress GATA6 expression by binding directly to its 3′-UTR region, which in turn causes a reduction in Lgr5 gene expression. Furthermore, we showed that ectopic expression of miR-363 suppresses the tumourigenicity of colorectal cancer cells and that overexpression of either GATA6 or Lgr5 could restore tumourigenic potential in cells expressing miR-363. In the latter experiments, restoration of tumourigenicity of cells overexpressing miR-363 was more efficiently induced by overexpression of GATA6 compared with Lgr5. This result is consistent with the fact that exogenous expression of Lgr5 was weaker than GATA6 in these experiments. Furthermore, we have observed that GATA6 transactivates many target genes other than Lgr5 that are important for tumourigenesis. It has been reported that miR-363 is also downregulated in the head and neck squamous carcinoma, resulting in the upregulation of podplanin ( PDPN ), a target gene that promotes cell migration and invasion [38] . However, we could not detect the expression of PDPN in DLD-1 or HT29 cells. We found that miR-363 regulates GATA6 protein levels, but not its mRNA levels. miRNAs generally inhibit protein synthesis by repressing translation and/or by causing destabilization of target mRNAs [39] , [40] . It is well known that miRNAs do not always induce both translational repression and mRNA destabilization. Some miRNA targets are very sensitive to degradation while others are mainly repressed translationally without marked destabilization. Thus, miR-363 appears to induce translational repression of GATA6 without inducing its mRNA degradation. The mechanism by which miRNAs induce translational repression has long been the subject of controversy. For example, it has been reported that miRNAs target initiation of translation, whereas it has also been reported that miRNAs inhibit various postinitiation steps. It remains to be investigated whether reported discrepancies are due to different experimental approaches or whether miRNAs can control translation by multiple mechanisms. miR-363 is derived from the miR-106a-363 cluster (miR-106a, miR-18b, miR-20b, miR-19b-2, miR-92a-2 and miR-363) on chromosome X. Moreover, this cluster is homologous to the miR-17-92 cluster (miR-17, miR-18a, miR-19a, miR-20a, miR-19b-1 and miR-92a-1), which is frequently upregulated in many tumours. In addition, the seed sequence of miR-363 is identical to those of miR-92a and miR-92b, which are overexpressed in solid tumours and leukaemia [41] , [42] , [43] . However, we found no significant differences in the expression levels of miR-92 between intestinal adenomas and normal tissues in Apc Min/+ mice. In conclusion, our study suggests that the miR-363-GATA6-Lgr5 pathway is critical for colorectal tumourigenesis. Consistent with this notion, recent studies have shown that gene fusions involving R-spondin family members, ligands for Lgr5, are observed in 10% of colon cancer and are mutually exclusive with mutations in APC and β-catenin [44] . Thus, we envision that the miR-363-GATA6-Lgr5 pathway could be a promising target for the therapy of colorectal tumours. Cell culture and plasmid transfection DLD-1 and HT29 cells (American Type Culture Collection, ATCC) were cultured in RPMI1640 medium supplemented with 10% fetal calf serum (FCS). RKO cells (ATCC) were cultured in minimum essential medium (MEM) supplemented with 10% FCS, MEM NEAA and Sodium pyruvate (GIBCO). HPAECs (TaKaRa) were cultured in EGM-2 medium (Cambrex) supplemented with dimerized Fibroblast Growth Factor, EGF, vascular endothelial growth factor, insulin-like growth factor 1 and 2% fetal bovine serum (FBS). 293FT cells (Invitrogen) were cultured in DMEM supplemented with 10% FCS. Plasmids were transfected into cells using Lipofectamine 2000 (invitrogen). Antibodies Rabbit polyclonal antibody to GATA6 (sc-9055), Lgr5 (ab75850) and α-actin (A2066) were from Santa Cruz, Abcam and Sigma, respectively. Rabbit polyclonal antibody to lysozyme (A0099) was obtained from Dako Cytomation. Mouse monoclonal antibody to α-tubulin (CP06) and Integrin β4 (611232) were from Oncogene Research and BD Biosciences, respectively. Mice and clinical samples Mouse experiments were approved by the Ethics Committee of the Institute of Molecular and Cellular Biosciences, The University of Tokyo and were performed according to ‘the Guidelines for Proper Conduct of Animal Experiments’ provided by the Science Council of Japan. C57BL/6J- Apc Min/+ mice were obtained from The Jackson Laboratory (Bar Harbor, ME, USA). BALB/CA nude mice were obtained from CLEA Japan (Tokyo, Japan). Following informed consent, resected colon cancer specimens were obtained from patients who underwent surgical treatment at the Department of Surgical Oncology, The University of Tokyo Hospital as approved by the Institutional Review Board. Transfection of siRNAs and microRNA precursor and inhibitor Stealth siRNA duplexes (Invitrogen), synthetic microRNA (miR-363 Pre-miR, Ambion) and microRNA inhibitor (miR-363 Anti-miR, Ambion) were transfected using Lipofectamine RNAiMAX (Invitrogen) 24 h after seeding. Validated Stealth negative control RNAi duplex with medium GC content (Invitrogen) and Pre-miR and Anti-miR negative control (Ambion) were used as a control. Sequences of siRNAs are listed in Supplementary Table 1 . Biotinylation of cell surface proteins In Fig. 4e , cells were washed with ice-cold PBS+ three times and biotinylated with 1% of EZ-Lnink Sulfo-NHS-LC-Biotin (Thermo) in PBS+ at 4 °C for 20 min. Biotin-labeled cells were washed with 50 mM glycin/PBS+ three times and lysed in RIPA buffer (1% NP-40, 0.5% DOC, 0.1% SDS, 20 mM Tris·HCl pH 7.5, 50 mM NaF, 150 mM NaCl, 1 mM DTT). Lysates were incubated with Streptavidin Agarose Resin (Thermo) for 16 h at 4 °C. After three washes with RIPA buffer and once with PBS+, isolated proteins were separated by SDS–polyacrylamide gel electrophoresis followed by immunoblotting analyses with anti-Lgr5 antibody (1:1,000 dilution). Histology and immunohistochemistry Formalin-fixed, paraffin-embedded sections of surgical specimens from patients and DLD-1 tumours were deparaffinizaed and rehydrated. Tumour sections were stained with hematoxylin and eosin (H/E), Periodic acid Schiff staining system (Sigma) or the indicated antibody. Antigen retrieval was performed using microwave in 10 mM sodium citrate buffer. Sections were treated with 3% goat serum and incubated with primary antibody (anti-lysozyme; 1:400 dilution). Diaminobenzidine staining procedure was performed using the VECTORSTAIN ABC system (Vector Laboratories). Hematoxylin was used for counterstaining. Tumourigenesis assays DLD-1 or HT29 cells infected with a lentivirus were suspended in PBS with equal volume of matrigel (BD Biosciences) and were subcutaneously injected (1 × 10 3 cells per mouse) into 7-10-week-old male nude mice. Tumour appearance was evaluated using a caliper and the tumour volume was calculated according to the formula (V=π/6 × [ L × W 2 ]), where V=volume, L =length and W =width (length is greater than width). Cell proliferation assays and colony formation assays DLD-1 cells were seeded in six-well plates at 1.0 × 10 5 cells per well and cell proliferation was measured by counting cell number every 24 h. For colony formation assays, a base layer was made by mixing 1% soft agar (BD) and equivalent 2 × RPMI1640 medium and pouring 500 μl of this into six-well plates. Dispersed DLD-1 cells were suspended in RPMI1640 medium containing 0.33% soft agar and seeded upon the base layer at a density of 500 cells per well. Plates were maintained at 37 °C in a humidified incubator. After 2 weeks, the number of colonies was assessed by counting under a microscope: ~70% of control cells formed colonies. All experiments were conducted in triplicate. RNA isolation and qRT–PCR Total RNA was isolated from cultured cells, mice and human tissues using NucleoSpin RNA II (MACHEREY-NAGEL) and TRIsure reagent (BIOLINE). First-stranded complementary DNA was synthesized using PrimeScript RT Master Mix (TAKARA). Quantitative reverse transcriptase (qRT–PCR) was performed in duplicate by the LightCycler 480 Real-Time PCR System (Roche). Total RNA containing miRNA was isolated using miRNeasy Mini Kit (QIAGEN). For qRT–PCR analysis of miRNAs, Mir-X miRNA First-Strand Synthesis Kit (Clontech) was used. Primer sequences are listed in Supplementary Table 1 . Immunoblotting analyses Cells or tissue samples were lysed in RIPA buffer (1% NP-40, 0.5% DOC, 0.1% SDS, 20 mM Tris·HCl pH 7.5, 50 mM NaF, 150 mM NaCl, 1 mM DTT). After centrifugation, the supernatants were resolved by SDS–polyacrylamide gel electrophoresis, transferred to a polyvinylidene difluoride membrane filter (Millipore) and analysed by immunoblotting using horseradish peroxidase-conjugated secondary antibodies. Super Signal West Pico Chemiluminescent Substrate (Thermo Fisher Scientific) and ECL Plus Western Blotting Detection System (GE Healthcare) were used as reaction substrates for chemiluminescent. Dilutions of primary antibodies were as follows: anti-GATA6, 1:500; anti-Lgr5, 1:1,000; anti-α-actin, 1:1,000; anti-α-tubulin, 1:1,000; anti-Integrin β4, 1:1,000. Full-length images of immunoblots are shown in Supplementary Fig. 3 . Construction of luciferase reporter vectors The promoter regions of Lgr5 were amplified by PCR using corresponding-specific primers and cloned into pGL3-basic (Promega). The 3′-UTR fragment of human GATA6 was amplified by PCR and cloned into the 3′ end of the Renilla luciferase sequence in pRL-TK vector (Promega). The mutant construct Mut 3′-UTR, which contains a mutated miR-363 seed sequence in the GATA6 3′-UTR were generated by site-directed mutagenesis. Luciferase assays Luciferase assays were performed using the Dual Luciferase Assay System (Promega). pRL-TK and pGL3-SV40 were used as internal controls for the experiments shown in Figs 2 and 4 , respectively. ChIP assays ChIP assays were performed according to the manufacturer’s instructions (Upstate). Briefly, DLD-1 cells were fixed with 1% formaldehyde for 10 min at room temperature and treated with 0.125 M glycine for 5 min. Cross-linked chromatin was resuspended in sonication buffer (50 mM Tris-HCl, 10 mM EDTA, 1% SDS), sheared into fragments with average length of ~600 bp. Immunoprecipitaion was performed using anti-GATA6 antibody (10 μg ml −1 ). Primer sequences for quantitative PCR are listed in Supplementary Table 1 . Microarray analysis Microarray analysis of gene expression in DLD-1 cells infected with an lentivirus expressing an shRNA targeting Lgr5 or GATA6 or control shRNA were performed using Agilent one-color microarrays (Agilent Whole Human Genome Microarray 4 × 44K chips (Agilent Technologies)). Normalization and analysis of the data were performed using Gene Spring version 11.5.1 (Agilent Technologies). Genes downregulated >1.7-fold by Lgr5 knockdown and those downregulated >twofold by GATA6 knockdown were identified as ‘LGR5 signature’ and ‘GATA6 signature’, respectively. The significance of the overlap between the Lgr5 signature and GATA6 signature was calculated by the hypergeometric distribution [45] . The data derived from microarray analysis have been deposited in the Gene Expression Omnibus (GEO) database under accession code GSE32987 . Generation and infection of a lentivirus expressing an shRNA Lentiviral vector (CS-Rfa-CG) expressing an shRNA or a miRNA sequence driven by the H1 promoter was generated using Gateway Technology (Invitrogen) and transfected with the packaging vectors pCAG-HIV-gp and pCMV-VSV-G-RSV-Rev into 293FT cells. The expression of lentiviral FLAG-tagged GATA6 or Lgr5 or control LacZ is under the cytomegalovirus (CMV) promoter. All plasmids were kindly provided by H. Miyoshi (RIKEN BioResource Center, Japan). Virus supernatants were purified by ultracentrifugation and dissolved in PBS. DLD-1 and HT29 cells were infected with a lentivirus at 37 °C for 1 h. Infected cells were cultured for more than 5 days before use in experiments. Oligonucleotide sequences of shRNA are listed in Supplementary Table 1 . Statistical analyses Statistical analysis was performed using the Mann–Whitney U -test and the Student’s t -test. A P -value <0.05 was considered to be statistically significant. Accession codes: The microarray data have been deposited in the GEO database under accession code GSE32987 . How to cite this article: Tsuji, S. et al. The miR-363-GATA6-Lgr5 pathway is critical for colorectal tumourigenesis. Nat. Commun. 5:3150 doi: 10.1038/ncomms4150 (2014).